Persistence of pressure patterns over North America and the North Pacific since AD 1500 Changes in moisture delivery to western North America are largely controlled by interrelated, synoptic-scale atmospheric pressure patterns. Long-term records of upper-atmosphere pressure and related circulation patterns are needed to assess potential drivers of past severe droughts and evaluate how future climate changes may impact hydroclimatic systems. Here we develop a tree-ring-based climate field reconstruction of cool-season 500 hPa geopotential height on a 2° × 2° grid over North America and the North Pacific to AD 1500 and examine the frequency and persistence of preinstrumental atmospheric pressure patterns using Self-Organizing Maps. Our results show extended time periods dominated by a set of persistent upper-air pressure patterns, providing insight into the atmospheric conditions leading to periods of sustained drought and pluvial periods in the preinstrumental past. A striking shift from meridional to zonal flow occurred at the end of the Little Ice Age and was sustained for several decades. The position of the mid-latitude storm track, which represents the primary large-scale moisture-delivery pathway to North America, is closely connected to the strength and position of upper-atmosphere pressure features such as the Pacific subtropical high and the Aleutian low [1] . Changes in these synoptic pressure features have been linked to global-scale oscillations in coupled ocean–atmosphere systems (particularly the El Niño–Southern Oscillation (ENSO) system) [2] , [3] and to Northern Hemisphere wave-train disturbances such as those described by the Pacific North American (PNA) pattern [4] . Shifts in the dominance of certain synoptic-scale atmospheric features have occurred over the instrumental period and influenced drought and flood regimes in western North America, including the early 20th century pluvial period and the devastating droughts of the 1930s and 1950s (ref. 5 ). Records from tree rings and other paleoclimate proxies have provided insight into the range of variability in the hydroclimatic system beyond the relatively short instrumental record. One of the most important findings in water-limited western North America is that there have been periods of severe and sustained drought in the preinstrumental past exceeding known droughts from the instrumental record [6] . The cause of these droughts is thought to be sustained shifts in moisture delivery processes linked to changes in ocean–atmosphere systems, particularly ENSO [6] . While many droughts are synchronous with La Niña events, others are not and require additional explanation such as the inclusion of North Pacific influences [3] . Long-term pressure data derived from the tree-ring record can be used to extend our understanding of these shifts in moisture-delivery processes by allowing an assessment of the frequency and persistence of certain circulation patterns and their variability through time. Although there have been numerous reconstructions of teleconnection indices, relatively few studies have engaged in synoptic dendroclimatology as a way to link tree growth with large-scale climate delivery systems through a focus on pressure patterns [7] . Pressure itself does not limit tree growth, but seasonal pressure anomalies reflect large-scale, persistent perturbations in climate [8] and are associated with the suite of variables that do control growth, including temperature, moisture, wind and cloud cover [7] , [9] . Past research comparing pressure data with tree-ring growth over the instrumental time period found that variations in pressure accounted for more variance in growth than did single climate variables such as temperature or precipitation, likely due to the multivariate climate controls on growth that are reflected in pressure fields [7] . Pressure anomalies in the upper atmosphere can persist for years to decades and influence temperature, precipitation and storm tracks over North America [9] . Extending the record of these anomalies would allow for a better understanding of the drivers of past climate conditions. This has become particularly important for future climate change forecasting and planning, as ongoing changes in atmospheric circulation due to anthropogenic forcing have already been identified [9] . Here, we use regularized expectation maximization with ridge regression (RegEM-ridge) [10] , [11] to develop a spatial reconstruction of cool-season, 500 hPa geopotential height (GPH) anomalies since AD 1500. We then investigate dominant synoptic climate patterns embedded within this reconstruction using Self-Organizing Maps (SOM). Our findings, which show extended time periods dominated by a set of persistent upper-air pressure patterns over the 511-year record, provide insight into the atmospheric conditions associated with distinctive terrestrial hydroclimate conditions in the preinstrumental past and suggest that the end of the Little Ice Age (LIA) was marked by an abrupt transition from strong meridional to zonal flow. Reconstructed atmospheric pressure RegEM-ridge [10] , [11] , which utilizes covariance within and between the instrumental and proxy data to iteratively impute missing values in the full data matrix, has been applied in previous paleoclimate reconstructions [12] , [13] and has demonstrated skill with the datasets used in this study [14] . Our reconstruction, developed using tree-ring data from the International Tree-Ring Data Bank (ITRDB; Fig. 1 and Methods) and NCEP/NCAR Twentieth Century Reanalysis V2 climate data (20CR2) provides cool-season (October–March), 500 hPa GPH anomalies back to AD 1500 on a 2° × 2° grid over western North America and the northeastern Pacific Ocean. The 500 hPa level has been widely used in the study of atmospheric circulation due the strength of teleconnection patterns at this height [4] . The October–March cool season is a time of pronounced teleconnection influence [4] and a vital period for moisture delivery to western North America [1] , [2] . The seasonal climate signal reflected in tree growth varies depending on geographic location, elevation and species [15] . Cool-season climate conditions have a strong influence on tree growth across a variety of climate zones due to effects on processes such as cambial activation, root mortality, xylem embolisms and soil moisture recharge [15] , [16] , [17] . The GPH reconstruction model demonstrates skill throughout the spatial domain as assessed by standard climate field reconstruction validation metrics ( Fig. 2 ). 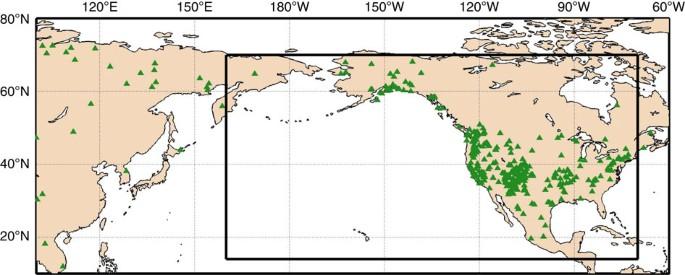Figure 1: Spatial domain of GPH reconstruction and tree-ring site locations. Cool-season (October–March) 500 hPa GPH anomalies were reconstructed on a 2° × 2° grid over 14°N–70°N latitude and 160°E–70°W longitude (inner box) using ITRDB tree-ring sites correlated with GPH at a 0.001 significance level (green triangles) within the spatial domain bounded by 10°N–80°N latitude and 100°E–60°W longitude (outer box). Figure 1: Spatial domain of GPH reconstruction and tree-ring site locations. Cool-season (October–March) 500 hPa GPH anomalies were reconstructed on a 2° × 2° grid over 14°N–70°N latitude and 160°E–70°W longitude (inner box) using ITRDB tree-ring sites correlated with GPH at a 0.001 significance level (green triangles) within the spatial domain bounded by 10°N–80°N latitude and 100°E–60°W longitude (outer box). 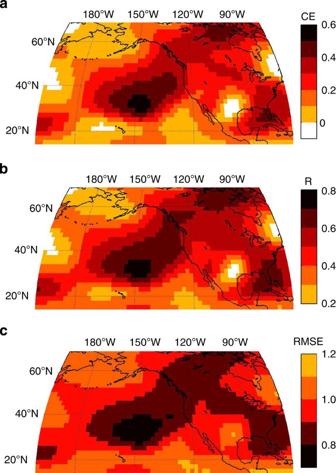Figure 2: Spatial validation metrics for the RegEM-ridge reconstruction model. (a) coefficient of efficiency (CE), where values of CE can range from −∞ to 1 and any CE greater than zero (shaded areas) indicates predictive skill. (b) Pearson correlation coefficient (R) between the predicted and observed data; all shaded grid cells are significant at or above the 95% confidence level. (c) root mean squared error (RMSE). Metrics of model skill were assessed using a leave-decade-out cross-validation approach over the 1872–1971 time period. Full size image Figure 2: Spatial validation metrics for the RegEM-ridge reconstruction model. ( a ) coefficient of efficiency (CE), where values of CE can range from −∞ to 1 and any CE greater than zero (shaded areas) indicates predictive skill. ( b ) Pearson correlation coefficient ( R ) between the predicted and observed data; all shaded grid cells are significant at or above the 95% confidence level. ( c ) root mean squared error (RMSE). Metrics of model skill were assessed using a leave-decade-out cross-validation approach over the 1872–1971 time period. Full size image Dominant synoptic climate patterns SOM, an unsupervised, artificial neural network approach [18] , [19] , was applied to the reconstructed data to analyse the frequency and persistence of atmospheric pressure patterns and their changes through time. The SOM technique organized the 511-year GPH dataset into a two-dimensional 3 × 5 grid topology of statistically distinguishable synoptic circulation patterns, or ‘nodes’ ( Fig. 3 ). Each of the 15 nodes represents a theoretical GPH pattern (rather than a composite of cases) based on the underlying data distribution within the input dataset. The primary differences among the GPH anomaly patterns ( Fig. 3 ) are the strength and position of the Aleutian low and the placement and degree of troughing or ridging over North America. Within the SOM organizational structure, there is a transition across columns 1 through 5 from a weak Aleutian low to a deep Aleutian low and from troughing over North America to ridging. Down through the three rows, there is a transition in strength and position of GPH anomalies, from patterns with relatively weak anomalies in row 1 to stronger anomalies in row 3. 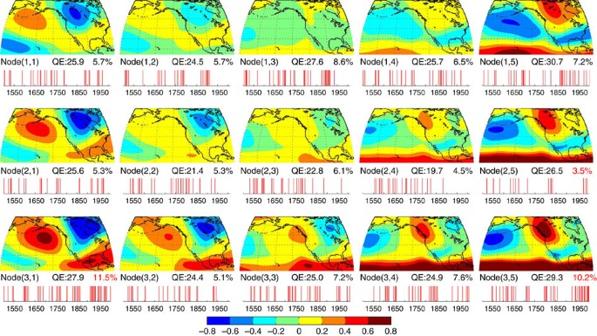Figure 3: Spatial and temporal distribution of GPH anomalies for AD 1500–2010. Maps show the spatial distribution of standardized GPH anomalies associated with the 15 SOM-classified node patterns. Individual years mapping to each node are shown with a present/absent bar graph time series below each map. Text between maps and time series indicates (left-to-right): nodes numbered as (row, column); average quantization error (QE) between the input years and each master node; and the pattern frequency (% of years) for the entire period mapping to each node. Frequencies that are above or below the expected range (95% confidence level; see Methods) are in red. Figure 3: Spatial and temporal distribution of GPH anomalies for AD 1500–2010. Maps show the spatial distribution of standardized GPH anomalies associated with the 15 SOM-classified node patterns. Individual years mapping to each node are shown with a present/absent bar graph time series below each map. Text between maps and time series indicates (left-to-right): nodes numbered as (row, column); average quantization error (QE) between the input years and each master node; and the pattern frequency (% of years) for the entire period mapping to each node. Frequencies that are above or below the expected range (95% confidence level; see Methods) are in red. Full size image These differences in mean upper-air pressure would result in changes to regional atmospheric flow patterns and storm-track trajectories. Overall, the weaker anomalies in row 1 suggest zonal flow patterns, transitioning to stronger meridional flow patterns through rows 2 and 3. Between rows 1 and 3, the ridge–trough pattern characteristic of PNA+ (columns 4 and 5) shifts to the west, while the reverse pattern (columns 1 and 2) shifts to the east ( Fig. 3 ). Changes in the position of the trough and ridge axes, which alter the spatial distribution of temperature and precipitation [5] , have important implications for terrestrial climate conditions. The transition in anomaly patterns across columns suggests a shift in the westerly storm track from more northerly flow in column 1 to increasingly southerly flow in column 5 ( Fig. 3 ). Columns 1 and 5 are strongly indicative of La Niña and El Niño conditions, respectively. On the basis of the instrumental record of ENSO, the La Niña-type GPH anomaly patterns (column 1) would likely be associated with a westward retraction of the East Asian jet stream and a bifurcated or northerly shift of the storm track across North America, while the El Niño-like patterns (column 5) would be associated with an enhanced East Asian jet stream and a storm track shifted south. Columns 2–4 represent transitions between these two extremes, including ENSO-neutral conditions. Circulation changes through time The placement of archetypal nodes that span the continuum of data allow SOM to capture non-linear aspects of the data and to operate without needing to conform to a specific predefined data distribution [18] , [19] . This is particularly relevant when dealing with paleoclimate, when dominant patterns may have differed from the instrumental period; however, there is still the potential for ‘no analog’ paleoclimate conditions that lie outside the instrumental data domain [20] . Each input value to the SOM (here, the yearly spatial grids of cool-season GPH anomalies) maps to the node with the lowest error, allowing analysis of frequency of occurrence through time [19] . The overall frequency of pattern occurrence is highly variable and ranges from 3.5 to 11.5%; three of the 15 nodes have frequencies that are significantly higher or lower than the expected value of 6.7% ( Fig. 3 ). Over the 511-year record, there have been sustained shifts in the prevalence of pressure patterns over time ( Figs 4 and 5 ). To emphasize changes across the SOM two-dimensional structure, we calculated the number of occurrences of each node (grouped by row and column) within 25-year moving windows, with statistical significance tested using a series of first-order Markov chain simulations [21] . Node assignments were further evaluated through comparison with an ensemble of plausible preinstrumental GPH fields generated using a suite of synthetic tree-ring records in a pseudoproxy experiment (PPE) [22] ( Figs 4 and 5 and Supplementary Tables 1 and 2 ). The most dramatic GPH pattern shift occurred following the end of the LIA (~AD1450–1850), when a 40-year period (1810s to 1850s) dominated by meridional flow (row 3) ended with a sharp transition to zonal flow (row 1) that was sustained for approximately 50 years (1860s to 1910s; Fig. 5 ). Beginning in the early 1900s, there was a slow transition back to persistent meridional flow (row 3). 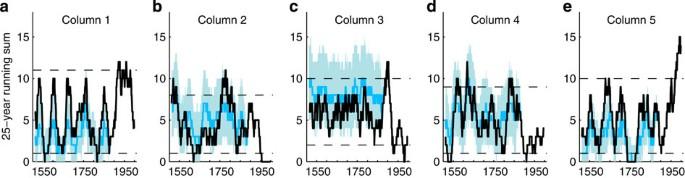Figure 4: Persistence of GPH anomaly patterns over time in SOM columns. Number of years within a 25-year moving window assigned to each SOM node (thick black lines) and grouped by SOM columns 1–5 (panelsa–e). 95% confidence intervals (dashed black lines) calculated using Markov Chain simulations. Results based on alternative realizations of the reconstructed GPH field generated using a 1,000-member PPE ensemble are shown with a blue line (median ensemble member) and blue shading (ensemble members falling within the 2.5th–97.5th percentiles). Figure 4: Persistence of GPH anomaly patterns over time in SOM columns. Number of years within a 25-year moving window assigned to each SOM node (thick black lines) and grouped by SOM columns 1–5 (panels a – e ). 95% confidence intervals (dashed black lines) calculated using Markov Chain simulations. Results based on alternative realizations of the reconstructed GPH field generated using a 1,000-member PPE ensemble are shown with a blue line (median ensemble member) and blue shading (ensemble members falling within the 2.5th–97.5th percentiles). 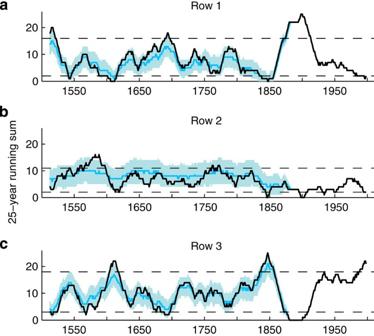Figure 5: Persistence of GPH anomaly patterns over time in SOM rows. Number of years within a 25-year moving window assigned to each SOM node (thick black lines) and grouped by SOM rows 1–3 (panelsa–c). 95% confidence intervals (dashed black lines) calculated using Markov Chain simulations. Results based on alternative realizations of the reconstructed GPH field generated using a 1,000-member PPE ensemble are shown with a blue line (median ensemble member) and blue shading (ensemble members falling within the 2.5th–97.5th percentiles). Full size image Figure 5: Persistence of GPH anomaly patterns over time in SOM rows. Number of years within a 25-year moving window assigned to each SOM node (thick black lines) and grouped by SOM rows 1–3 (panels a – c ). 95% confidence intervals (dashed black lines) calculated using Markov Chain simulations. Results based on alternative realizations of the reconstructed GPH field generated using a 1,000-member PPE ensemble are shown with a blue line (median ensemble member) and blue shading (ensemble members falling within the 2.5th–97.5th percentiles). Full size image The end of the LIA in the mid-1800s has been identified as a period of fundamental change in atmospheric circulation [23] , [24] , and major climatic shifts during this period have been documented in ice cores, lake cores and tree rings [25] . This change has been attributed to a major reorganization of Pacific Ocean circulation [23] , which may be related to an increased connection between the northern and tropical Pacific after the mid-1800s (ref. 26 ) or between the North Pacific and North Atlantic Oceans [24] . Multiple studies have indicated that the end of the LIA corresponded to reduced North Pacific decadal forcing [9] , [23] , [27] . The end of the LIA may also represent a shift from decadal variability to interannual ENSO mode after 1850 (refs 9 , 23 ), with a possible return to decadal variability following the 1976 North Pacific regime shift [23] . The El Niño (column 5) and La Niña (column 1) SOM patterns indicate multidecadal oscillations before the 1900s ( Fig. 4 ). On the basis of the GPH anomaly patterns ( Fig. 3 ), the striking shift in dominant atmospheric patterns at the end of the LIA ( Fig. 5 ) likely represents a shift from highly meridional to zonal flow. Ice core evidence suggests that the LIA was a period of increased meridional flow [28] , [29] , and historical records indicate a period of particularly intense meridional circulation in the 1840s (ref. 30 ). The climatic shifts at the end of the LIA may represent a weakening of trade winds over the Pacific [25] and a shift from meridional flow to zonal flow [8] , [25] . This reconstruction supports previous research [31] , [32] suggesting that the majority of the LIA was a period of fluctuating climate conditions rather than a sustained, uniform climate period: before the 1800s, the LIA was characterized by variability across all nodes, although there have been other periods of sustained and persistent GPH anomaly patterns on decadal time scales. Since the early 1900s, there has been a transition back from persistent zonal (row 1) patterns to the dominance of meridional (row 3) patterns ( Fig. 5 ). Identified shifts in the frequencies and magnitudes of synoptic features can help identify and describe regime shifts in climate and can be useful descriptors of climate variability and change. Understanding ‘steps’ in climate is important for explaining past events and for future planning, particularly in light of the strong links between atmospheric circulation and hydrologic variability. Evidence from climate models suggests that future regional changes in hydroclimate will depend on multiple drivers of atmospheric moisture transport [6] . Although uncertainties still exist, observations and modelling experiments point to an increase in the frequency and intensity of El Niño, with an associated southward shift and intensification of the subtropical jet stream, an enhanced PNA pattern and an increase in winter and spring storms across much of the U.S. and western Canada [33] , as well as a decrease in zonal flow and weakened westerlies into North America [34] . This reconstruction, which allows dominant atmospheric circulation features of the 20th century to be compared with earlier time periods, indicates that over the past several decades, GPH anomaly patterns have persistently clustered in configurations that mirror observed and modelled climate changes, such as the positive trend in the instrumental PNA index [35] ( Figs 4 and 5 ). These trends in synoptic circulation patterns have important implications for storminess, snowpack and streamflow in North America [33] , [34] , [35] , and the dominant pressure patterns characterized here will allow for an examination of associated terrestrial climate impact patterns in future research. Climate field reconstruction model Raw tree-ring widths within the spatial domain bounded by 10°N to 80°N latitude and 100°E to 60°W longitude were obtained from the ITRDB ( Fig. 1 , www.ncdc.noaa.gov/paleo/treering.html ), detrended with a cubic spline two-thirds the length of each individual series, and combined to form site chronologies. This collection was screened to remove duplicate tree-ring series, series with missing data, and series that did not span at least the 1800–1971 time period. Retaining chronologies with an end date of 1971 or later retained >90% of the available chronologies while still allowing for a robust 100-year calibration interval. Remaining chronologies underwent significance pre-screening for inclusion into the model: only chronologies correlated at a 0.001 significance level with at least one climate grid cell were retained in the model. Monthly mean 500 hPa GPH values from 20CR2 (ref. 36) [36] , spanning 1871–2010 at a 2.0° × 2.0° resolution, were converted to cool-season (October–March) anomalies (assigned to the ending year of the season) and used to calibrate the reconstruction model. The spatial domain for the GPH reconstructed grid is 14°N-70°N; 160°E-70°W ( Fig. 1 ). We used RegEM-ridge [11] , [14] to reconstruct cool-season (October–March) 500 hPa GPH anomalies. We assessed model skill using a cross-validation approach wherein 10-year blocks of GPH data were successively withheld and the model was standardized and calibrated using all remaining values, which were then used to estimate the withheld values. This process was repeated through each of the ten decades in the series. To increase independence of each decadal block, the five years of data preceding and following each decade were not used for calibration of the model. Following model validation, both proxy and instrumental data were standardized over the calibration period (1872–1971) for use with the reconstruction model and combined in the input data matrix. We applied a stepwise approach [12] , [13] in which the reconstruction was completed by century and the imputed values were incorporated in the data matrix as the RegEM algorithm was applied to successively older segments. Synoptic climatological analysis We used the SOM Toolbox (freely available at http://www.cis.hut.fi/somtoolbox ) for synoptic climatological analysis of the frequency and persistence of atmospheric pressure patterns and their changes through time. SOM is a neural network approach that treats data as a continuum rather than discrete classes and can be used to objectively identify patterns through the use of an iterative clustering algorithm [18] . The SOM technique requires the user to make an a priori decision concerning the number of nodes ( K ). Here, we use the false discovery rate technique [21] , [37] to determine the value of K +1, or the point at which one or more pairs of SOM node patterns become statistically indistinguishable at the 95% confidence level. For each tested value of K (2 through 25), local two-sample t -tests are performed at each grid cell between data assigned to every possible pair of nodes. Given the large number of local tests, there is a high probability of ‘false discovery’ (an incorrect rejection of the null hypothesis). The false discovery rate test corrects for this by examining the distribution of local P -values resulting from each of the local t -tests [37] : where q is the global test level, p j is the P -value of the j th local t -test and K is the total number of grid cells for which a t -test is performed. If the P -value of any local t -test is smaller than predicted from the uniform distribution of local P -values (that is, satisfies the condition in equation (1)), then that test is considered significant and the two node pairs are considered statistically distinguishable [21] , [37] . Here, the maximum number of statistically distinct GPH patterns used 15 nodes; therefore, we use a 15-node master SOM, which ‘self-organized’ into a two-dimensional (3 × 5) grid topology. Each input value presented to the SOM (in this case, cool-season GPH anomaly fields from 1500 to 2010) is assigned to the best-matching node in such a way as to minimize the quantization error, based on the Euclidean distance between the input data and the master SOM [38] . The probability of any given year mapping to a particular node is P =1/ N , where N is the number of nodes. The expected frequency of occurrence ( F ) of any of the nodes over the entire period [38] at the 95% confidence level is given by: In this study, P =1/15 (6.7%); n =511 (number of years) and F =4.5–8.8% (95% confidence interval). We calculated 25-year running sums of node occurrence grouped by SOM column and row and assessed 95% confidence intervals using a series of Markov Chain simulations. Markov Chains were constructed by calculating a frequency matrix of transitions from one ‘state’ (row or column) in year t to another in year t+ 1, and we converted the frequency matrix into a transition probability matrix by dividing each element by its row sum [39] . Twenty-five year synthetic ‘chains’ were generated by randomly assigning the first year of each chain to one of the three rows (or one of the 5 columns) and then using the transition probability matrix to weight a random assignment of the remaining 24 years based on the ‘state’ of the previous year. For each chain, the number of occurrences of the rows and columns were calculated, and 95% confidence levels were defined as any 25-year period greater than the 97.5th or less than the 2.5th percentile of 10,000 synthetic chains [21] . Pseudoproxy comparison We evaluated the range of plausible preinstrumental GPH fields that could be generated from the available tree ring and 20CR2 data using a PPE [22] . One thousand sets of synthetic tree-ring observations (each set consisting of the same number of records and temporal coverage as the actual ITRDB dataset used in this study) were generated based on random draws from the multivariate normal distribution defined by the in-filled data matrix (GPH+proxy data) and estimated covariance matrix from the final RegEM-ridge model. These pseudoproxies were then substituted into the in-filled data matrix (in place of the tree-ring records), the covariance matrix was re-estimated and this updated covariance matrix was used to impute the missing preinstrumental GPH values using RegEM-ridge [11] , resulting in an ensemble of 1,000 plausible GPH fields covering the preinstrumental period (1500–1871). The annual GPH fields from each PPE were then assigned to nodes in the SOM and 25-year running sums of row and column occurrences were calculated using the same methods as in the previous reconstruction analysis ( Figs 4 and 5 ). We compared yearly SOM row and column assignments from the alternative GPH realizations produced by the PPE ensemble to those of the original GPH reconstruction and evaluated them against random occurrences using equation (2) ( Supplementary Tables 1 and 2 ). How to cite this article: Wise, E. K. and Dannenberg, M. P. Persistence of pressure patterns over North America and the North Pacific since AD 1500. Nat. Commun. 5:4912 doi: 10.1038/ncomms5912 (2014).